Three-dimensional controlled growth of monodisperse sub-50 nm heterogeneous nanocrystals The ultimate frontier in nanomaterials engineering is to realize their composition control with atomic scale precision to enable fabrication of nanoparticles with desirable size, shape and surface properties. Such control becomes even more useful when growing hybrid nanocrystals designed to integrate multiple functionalities. Here we report achieving such degree of control in a family of rare-earth-doped nanomaterials. We experimentally verify the co-existence and different roles of oleate anions (OA − ) and molecules (OAH) in the crystal formation. We identify that the control over the ratio of OA − to OAH can be used to directionally inhibit, promote or etch the crystallographic facets of the nanoparticles. This control enables selective grafting of shells with complex morphologies grown over nanocrystal cores, thus allowing the fabrication of a diverse library of monodisperse sub-50 nm nanoparticles. With such programmable additive and subtractive engineering a variety of three-dimensional shapes can be implemented using a bottom–up scalable approach. Nanocrystal engineering, design and fabrication of nanocrystals with desirable size, shape [1] , [2] , [3] , [4] , [5] , [6] , surface properties [7] and composition [8] , [9] is attracting growing interest due to its essential role in fundamental research and commercial relevance. Rare-earth-doped upconversion nanocrystals have recently emerged as the new generation of functional nanomaterials, because they exhibit exceptional optical, magnetic and chemical properties underpinning their diverse applications. In particular, alkaline rare-earth fluoride (AREF 4 ) nanocrystals [10] , [11] , [12] , including hexagonal-phase β-NaYF 4 , β-NaGdF 4 , β-NaNdF 4 or β-NaLuF 4 are used in full-colour displays [12] , [13] , photovoltaics [14] , security inks [15] , forensic science [16] , autofluorescence-free biomolecular sensing [17] , [18] , [19] , multimodal in vivo bio-imaging (fluorescence, magnetic resonance imaging, X-ray, SPECT and so on.) [20] and theranostics [17] , [21] , [22] , [23] . A trial-and-error approach is frequently used to produce nanoparticles with spherical, rod-like or other shapes [24] , [25] , [26] by varying dopant concentrations and/or constituent materials [27] , reaction time and temperature [28] , [29] , [30] , [31] . This random sampling of vast, multidimensional parameter space, needs to be done rationally, with proper understanding of the underpinning growth mechanisms. Here we find that oleate anions (OA − ), the dissociated form of oleic acid molecules (OAH), have variable, dynamic roles in mediating the growth of AREF 4 nanocrystals. This allows us to introduce a molecular approach to tailoring the shape and composition of AREF 4 nanocrystals. This new method is based on a selective epitaxial core–shell growth process in the presence of oleic acid, commonly used as a surfactant during the synthesis of β-AREF 4 nanocrystals [32] . Drawing inspiration from the recently discovered co-existence of oleic acid molecules (OAH) and their dissociated form, oleic acid ions (OA − ) in the binary systems of PbS [33] and PbSe nanocrystals [34] , we hypothesize that the change in the ratio of OA − to OAH could influence the interaction of these ligands with the particle surface and hence the resulting morphology. Our computational modelling ( Fig. 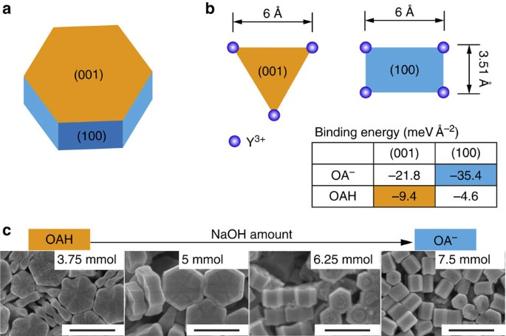Figure 1: Preferred molecular bonding models of OA−and OAH. (a) The schematic shape of aβ-NaYF4nanocrystal chosen as the core for directional epitaxial growth in this work. The hexagonal cylinder consists of the (001) facets at the ends and identical (100) and (010) facets around the cylinder sides. (b) The Y3+arrangements and binding energies (see insert table) of OAH and OA−on the most stable (001) and (100) facets. The Y3+atoms form equilateral triangles with a length of 6 Å in the relaxed (001) surface, while rectangles are observed in the (100) surface with a shorter length of 3.51 or 3.69 Å; (c) SEM characterization of submicron-sized nanocrystals synthesized using the hydrothermal route (detailed synthesis is included in the method; scale bar, 500 nm). 1 , Supplementary Figs 1–6 , Supplementary Notes 1 and 2 and Supplementary Table 1 ) and experimental results ( Figs 2 , 3 , 4 , Supplementary Figs 7–35 , Supplementary Tables 2 and 3 and Supplementary Notes 3–18 ) demonstrate that the preferential affinity of OAH and OA − to different crystalline facets dictates the formation of nanocrystals of different shape. Importantly, we demonstrate that the precise control over the shell thickness and the particle shape can be achieved by deliberately switching the passivation, additive and subtractive roles of these surfactants. Figure 1: Preferred molecular bonding models of OA − and OAH. ( a ) The schematic shape of a β -NaYF 4 nanocrystal chosen as the core for directional epitaxial growth in this work. The hexagonal cylinder consists of the (001) facets at the ends and identical (100) and (010) facets around the cylinder sides. ( b ) The Y 3+ arrangements and binding energies (see insert table) of OAH and OA − on the most stable (001) and (100) facets. The Y 3+ atoms form equilateral triangles with a length of 6 Å in the relaxed (001) surface, while rectangles are observed in the (100) surface with a shorter length of 3.51 or 3.69 Å; ( c ) SEM characterization of submicron-sized nanocrystals synthesized using the hydrothermal route (detailed synthesis is included in the method; scale bar, 500 nm). 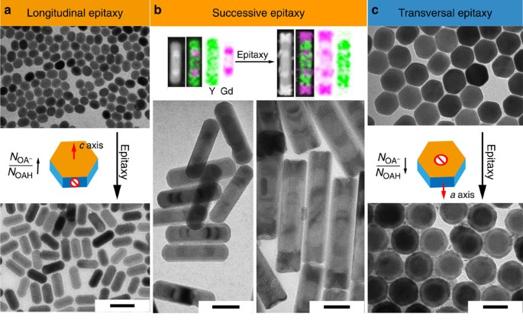Figure 2: Physical characterization of epitaxial growth of NaReF4NCs. (a) NaYF4core and homogenous NaYF4NCs after epitaxial growth of NaYF4in longitudinal direction with 0.5 mmol NaOH and 9.5 mmol OA at 310 °C for 1 h; (b) five-section and seven-section ‘bamboo-shaped’ NaYF4/NaGdF4NRs formed by successive heterogeneous growth of periodical shells of NaGdF4–NaYF4and NaGdF4–NaYF4–NaGdF4onto NaYF4core in the longitudinal direction, with 0.5 mmol NaOH and 0.4 mmol KOH and 9.5 mmol OA at 310 °C. Upper part of the panel shows elemental mapping of Y and Gd; (c) NaYF4core and heterogeneous NaYF4/NaGdF4NCs after epitaxial growth of NaGdF4in the transversal direction with 0.15 mmol NaOH and 19 mmol OA at 290 °C for 3 h; the dimensions of individual nanocrystal were analysed statistically and included in theSupplementary Figs 10, 20–24. Scale bar, 50 nm. Full size image Figure 2: Physical characterization of epitaxial growth of NaReF 4 NCs. ( a ) NaYF 4 core and homogenous NaYF 4 NCs after epitaxial growth of NaYF 4 in longitudinal direction with 0.5 mmol NaOH and 9.5 mmol OA at 310 °C for 1 h; ( b ) five-section and seven-section ‘bamboo-shaped’ NaYF 4 /NaGdF 4 NRs formed by successive heterogeneous growth of periodical shells of NaGdF 4 –NaYF 4 and NaGdF 4 –NaYF 4 –NaGdF 4 onto NaYF 4 core in the longitudinal direction, with 0.5 mmol NaOH and 0.4 mmol KOH and 9.5 mmol OA at 310 °C. Upper part of the panel shows elemental mapping of Y and Gd; ( c ) NaYF 4 core and heterogeneous NaYF 4 /NaGdF 4 NCs after epitaxial growth of NaGdF 4 in the transversal direction with 0.15 mmol NaOH and 19 mmol OA at 290 °C for 3 h; the dimensions of individual nanocrystal were analysed statistically and included in the Supplementary Figs 10, 20–24 . Scale bar, 50 nm. 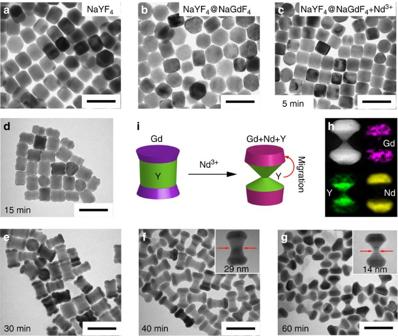Figure 3: Evolution of morphology and composition in migration growth. (a,b) NaGdF4growth along the longitudinal direction onto the ends of the NaYF4core; (c) transmission electron microscope image of the sample stopped 5 min after reacting with NaGdF4/NaYF4nanocrystals in the presence of Na+, K+, Nd3+, OA−and in the absence of F−at 310 °C, dissolution occurs first; (d–g) real-time monitoring of the epitaxial growth of NaNdF4along the longitudinal direction onto NaYF4–NaGdF4nanocrystals, involving the dissolution of NaYF4and NaGdF4from the transversal surfaces of the crystal and their subsequent re-growth onto the NaNdF4nanocrystals in the presence of Na+, K+, Nd3+, OA−and absence of F−ions at 310 °C. (h) HAADF-STEM image with elemental mapping results of the samples stopped after 60 min of reaction to confirm the distributions of Y3+, Gd3+, Nd3+ions within a single NaYF4/NaGdF4/NaNdF4nanocrystal. (i) schematic processes of dissolution of NaYF4/NaGdF4and the sequent epitaxial growth of NaNdF4in the longitudinal direction and the migration growth of F−, Y3+and Gd3+ions (scale bar, 100 nm). Full size image Figure 3: Evolution of morphology and composition in migration growth. ( a , b ) NaGdF 4 growth along the longitudinal direction onto the ends of the NaYF 4 core; ( c ) transmission electron microscope image of the sample stopped 5 min after reacting with NaGdF 4 /NaYF 4 nanocrystals in the presence of Na + , K + , Nd 3+ , OA − and in the absence of F − at 310 °C, dissolution occurs first; ( d – g ) real-time monitoring of the epitaxial growth of NaNdF 4 along the longitudinal direction onto NaYF 4 –NaGdF 4 nanocrystals, involving the dissolution of NaYF 4 and NaGdF 4 from the transversal surfaces of the crystal and their subsequent re-growth onto the NaNdF 4 nanocrystals in the presence of Na + , K + , Nd 3+ , OA − and absence of F − ions at 310 °C. ( h ) HAADF-STEM image with elemental mapping results of the samples stopped after 60 min of reaction to confirm the distributions of Y 3+ , Gd 3+ , Nd 3+ ions within a single NaYF 4 /NaGdF 4 /NaNdF 4 nanocrystal. ( i ) schematic processes of dissolution of NaYF 4 /NaGdF 4 and the sequent epitaxial growth of NaNdF 4 in the longitudinal direction and the migration growth of F − , Y 3+ and Gd 3+ ions (scale bar, 100 nm). 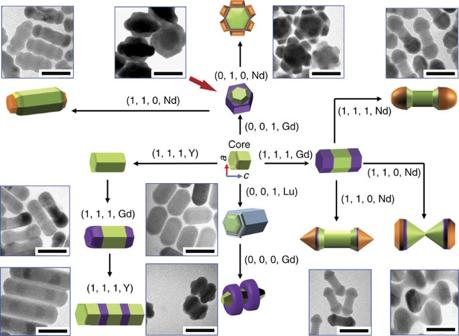Figure 4: Programmable routes for fabricating 3D nano-architectures. The four digital condition codes (R, T, F and RE) represent different reaction conditions where:R=0, represents a low ratio of OA−/OAH;R=1, represents a high ratio of OA−/OAH;T=0, where the temperature is at 290oC;T=1, where the temperature is at 310 °C;F=0, which designates the absence of anF−ion source;F=1, indicates the presence of anF−ion source; RE=Y, with a rare earth Y3+ion source; RE=Gd, with Gd3+ion source; RE=Lu, with a Lu3+source; RE=Nd, with Nd3+source. By combining these different growth processes into a synthesis procedure, a variety of complex NaREF4nanostructures are fabricated as shown in the transmission electron microscope images, including hourglass shaped NaYF4/NaGdF4/NaNdF4nanocrystals, NaYF4/NaGdF4/NaNdF4nano-flowers, NaYF4/NaLuF4co-axial nano-cylinders, NaYF4/NaLuF4/NaGdF4nanoscale spins with double rings, and NaYF4/NaGdF4/NaNdF4nano-dumbbells with smooth or sharp ends (scale bar, 50 nm). Full size image Figure 4: Programmable routes for fabricating 3D nano-architectures. The four digital condition codes (R, T, F and RE) represent different reaction conditions where: R =0, represents a low ratio of OA − /OAH; R =1, represents a high ratio of OA − /OAH; T =0, where the temperature is at 290 o C; T =1, where the temperature is at 310 °C; F =0, which designates the absence of an F − ion source; F =1, indicates the presence of an F − ion source; RE=Y, with a rare earth Y 3+ ion source; RE=Gd, with Gd 3+ ion source; RE=Lu, with a Lu 3+ source; RE=Nd, with Nd 3+ source. By combining these different growth processes into a synthesis procedure, a variety of complex NaREF 4 nanostructures are fabricated as shown in the transmission electron microscope images, including hourglass shaped NaYF 4 /NaGdF 4 /NaNdF 4 nanocrystals, NaYF 4 /NaGdF 4 /NaNdF 4 nano-flowers, NaYF 4 /NaLuF 4 co-axial nano-cylinders, NaYF 4 /NaLuF 4 /NaGdF 4 nanoscale spins with double rings, and NaYF 4 /NaGdF 4 /NaNdF 4 nano-dumbbells with smooth or sharp ends (scale bar, 50 nm). Full size image Computational modelling To quantify the surface coordination chemistry between β-NaYF 4 surface and OAH and OA − ligands, we performed first-principles calculations based on density functional theory using CASTEP (CAmbridge Serial Total Energy Package) [35] . As shown in Fig. 1b and Supplementary Fig. 1 , we treated the (001) and (100) planes of the β -NaYF 4 nanocrystals terminated with specific atomic arrangement as the most stable facets according to the calculated surface energies. Considering that the oxygen moiety in the ligands has a strong binding affinity to Y 3+ ions at the particle surface [36] , we modelled the interactions between the OAH and OA − molecules and the Y 3+ ions under a number of conditions, such as different adsorption configurations ( Supplementary Figs 2 and 3 and Supplementary Note 1 ), ligand chain length and ligand coverage ( Supplementary Figs 4 and 5 and Supplementary Note 2 ). The key conclusion from these simulations is that OA − preferentially binds to RE 3+ ions exposed on the (100) facet of the hexagonal fluoride nanocrystal, with a much higher binding energy (−35.4 eV) than on the (001) facet (−21.8 eV). It should be noted that the OAH molecule binds with a higher probability to the (001) facet than the (100) facet and has relatively small binding energies of −9.4 eV and −4.6 eV, respectively, on each of these facets ( Supplementary Table 1 ). Our charge analysis ( Supplementary Fig. 6 ) further indicates that such selective binding is attributed to the difference in the atomic arrangements of these two facets ( Fig. 1b ), giving rise to different charge transfer paths between the ligands and the surface ions. Controlled epitaxial growth direction The binding preferences of OAH and OA − molecules to different facets were first used to induce longitudinal epitaxial growth. We demonstrated ( Fig. 1c ) that sub-micrometre-sized NaYF 4 crystals of different aspect ratios could be prepared by tuning the concentration ratio of OA − to OAH in the hydrothermal synthesis system. As shown in Supplementary Fig. 7 , higher concentrations of OA − encourage epitaxial growth along a longitudinal direction. A similar effect was observed in the synthesis of sub-50 nm NaYF 4 nanoparticles prepared by a co-precipitation method. Figure 2a,b show that high concentration of NaOH leads to longitudinally grown nanoparticles because of a large concentration of passivating OA − ions on the (100) facets ( Supplementary Figs 8–10 ). The zeta potential of +20 mV for NaYF 4 nanocrystals after the removal of ligands ( Supplementary Fig. 11 ) shows that the RE 3+ cations are more abundant on the crystal surfaces than the F − ions. We further systemically studied other possible factors that could influence the epitaxial shell growth (experimental details in Supplementary Methods ), including the reaction temperature ( Supplementary Fig. 12 and Supplementary Note 3 ), the oleic acid concentration ( Supplementary Fig. 13 and Supplementary Note 4 ), the F − ion concentration ( Supplementary Fig. 14 and Supplementary Note 5 ) and the Na + concentration ( Supplementary Fig. 15 and Supplementary Note 6 ). From these results, we confirm that the ratio of OA − /OAH is a key factor that determines the epitaxial shell growth direction. However other parameters also have an effect on the growth speed or can change the OA − /OAH ratio that indirectly affects the direction of growth. To rule out the effect of OH − on longitudinal growth, we added sodium oleate as the sodium source instead of hydroxide and identical results were obtained ( Supplementary Fig. 16 and Supplementary Note 7 ). Supplementary Figures 17 and 18 further confirm that high ratio of OA − /OAH directs longitudinal deposition of heterogeneous shells (NaGdF 4 ) on the end surfaces of NaYF 4 core. Interestingly, subtractive growth (dissolution) is observed from their side (100) surfaces. This results in concurrent decrease of the core width from 26 to 18 nm, thus producing dumbbell-shaped nanocrystals ( Supplementary Note 8 ). Moreover, we found that the addition of KOH further accelerates longitudinal growth rate ( Supplementary Fig. 19 and Supplementary Note 9 ) due to a higher dissociation constant of KOH than NaOH, which increases the dissociation of OAH producing more OA − . With the aid of KOH, heterogeneous ‘bamboo-shaped’ nanorods (NRs) with sharp edges were formed in a stepwise manner with a length of up to 173 nm ( Fig. 2b , Supplementary Fig. 21 and Supplementary Note 10 ). The interesting one-dimension architecture of ‘bamboo-shaped’ NRs suggests that integrated multiple functionalities can be built. Thus our new platform enables rational design and facile synthesis of multiple sections of rare-earth-doped heterogeneous materials and investigation of their interactions and functions within a single integrated rod. We were also able to induce transversal epitaxial growth by increasing the amount of OAH and reducing the amount of NaOH. At a reaction temperature of 290 °C, the transversal growth was observed and NaGdF 4 rings of 7-nm-thick around the NaYF 4 cores formed without a measurable change in the longitudinal direction ( Fig. 2c , Supplementary Figs 23 and 24 and Supplementary Note 11 ). Notably, the dissolution of the (100) facets of the cores took place as well, and the width of the core was, again, reduced from 49 to 30 nm at both ends. The observed dissolution always occurred on the (100) facets in both cases of longitudinal and transversal growth. This is consistent with the strong chelating character of OA − on the (100) facet, and with the fact that NaYF 4 is dissolved faster than NaGdF 4 because NaYF 4 is comparably less energetically stable [12] . To shed more light on this issue, we provided more evidence in the Supplementary Fig. 25 and Supplementary Note 12 to show that the dissolution of core is caused by the thermal stability difference between core and shell materials in presence of OA − which leads to higher binding strength on the side surfaces. By comparing growth of NaTbF 4 as shell or NaYbF 4 as shell on a NaYF 4 core ( Supplementary Fig. 25 ), we demonstrate that the dissolution of the core requires the shell materials to have higher thermal stability than the core material. Larger difference of thermal stability between core and shell result in a higher dissolution rate. Controlled migration growth By combining the approaches of longitudinal and transversal growth and selective dissolution with consideration of lattice mismatch ( Supplementary Tables 2 and 3 ), we synthesized a variety of three-dimensional (3D) hybrid nanostructures ( Supplementary Figs 26–34 ). Figure 3 shows a typical example of real-time evolution of morphology and composition of the NaYF 4 /NaGdF 4 /NaNdF 4 NCs, including the dissolution process of the NaYF 4 /NaGdF 4 nanocrystals and subsequent longitudinal growth of NaNdF 4 . The dissolution of NaYF 4 /NaGdF 4 is initiated by the OA − adsorbed on the surface of the nanocrystals. The concomitant depletion of dissolved F − ions used for longitudinal growth of NaNdF 4 in the presence of high concentration of OA − facilitates the dissolution of NaYF 4 /NaGdF 4 nanocrystals and this, in turn, promotes longitudinal growth of NaNdF 4 . Following the dissolution of the Y 3+ and Gd 3+ ions from the surface of NaYF 4 –NaGdF 4 nanocrystals, these ions then participate in the epitaxial growth of NaNdF 4 nanocrystals, as evidenced by the elemental mapping ( Fig. 3h ). Moreover, our real-time sampling transmission electron microscope data further confirmed the underpinning mechanism ( Fig. 3a–g , Supplementary Figs 26–28 ). The size of nanocrystal core decreased significantly in the first 5 min, indicating that the dissolution rate of the nanocrystals is faster than their growth rate. After 15 min, new material started to form at the top and at the bottom ends of the core with simultaneous decrease of the nanocrystal core width. This observation rules out ‘surface mobility’ (‘atom diffusion’) as the possible driving force behind the formation of the final shell, otherwise it is expected that the dissolution of NaYF 4 and growth of NaNdF 4 would occur at the same time. The only mechanism which explains the shape of this nanocrystal is that the absence of F − source in the reaction solution at its beginning prevents growth of NaNdY 4 until the concentration of released F − source exceeds a certain threshold. Our control experiments ( Supplementary Fig. 29 and Supplementary Note 15 ) further support the mechanism of OA − -induced dissolution in which a firm bonding of the surfactant OA − to the surface RE 3+ cations is the main factor responsible for the removal of the surface crystalline layers (experimental details in Supplementary Methods ). As shown in Supplementary Fig. 29 , we applied transversal growth approach to first grow a layer of NaGdF 4 on the side surfaces of NaYF 4 core. We see that smaller mismatch of NaGdF 4 versus NaNdF 4 compared with the NaYF 4 versus NaNdF 4 fails to direct the transversal migration growth of the NaNdF 4 on the side surfaces of NaGdF 4 . Instead, dissolution occurs in the first 10 min of the reaction ( Supplementary Fig. 29a,b ) and both dissolution from the side surfaces and epitaxial growth of NaNdF 4 on the end surfaces of NaGdF 4 /NaYF 4 cores result in a thinner and longer nanocrystal. Guided by the principle that the ratio of OA − /OAH controls the direction of epitaxial shell growth, we further demonstrated (as shown in Supplementary Fig. 30 and Supplementary Note 16 ) that a low ratio of OA − /OAH at a lower temperature directs the migration growth along transverse direction. This enables the formation of heterogeneous NaYF 4 /NaGdF 4 /NaNdF 4 nanocrystals in the shape of a flower, although in this case the dissolution process on the side surfaces of nanocrystals is much less efficient because there are too few OA − ligands bound to RE 3+ cations on the (100) facet. Two additional experiments ( Supplementary Note 17 ) demonstrate that well established parameters, such as reagent concentration, can be further applied to fine-tune our programmable protocols for other types of heterogeneous nanocrystals. During the formation of hourglass-shaped nanocrystals, the decrease in the amount of Nd 3+ source is found to hinder the migration growth process and yield sharper tips ( Supplementary Fig. 31 ), whereas a supply of additional F − ions in the reaction increases the diameter of dumbbell ends with round tips ( Supplementary Fig. 32 ). Such level of fine tuning to grow progressively sharper tips may suggest future rational methods, for example to optimize tip-sensitive physical and biochemical properties of NRs. Figure 4 shows an array of heterogeneous NaREF 4 nanostructures synthesized by carrying out specific sequences of longitudinal, transversal growth, selective dissolution and directional migration growth of epitaxial shells in the presence of various OA − /OAH ratios. To the best of our knowledge, these sub-50 nm nanoparticles are the smallest 3D objects prepared by a bottom–up additive and subtractive process. To illustrate the application of this novel method we designed and synthesized multifunctional NaYF 4 /NaLuF 4 /NaGdF 4 heterogeneous nanocrystals with two NaGdF 4 rings on a NaLuF 4 /NaYF 4 NRs ( Supplementary Figs 33 and 34 and Supplementary Note 18 ). The hexagonal-phase NaYF 4 nanocrystal is an efficient luminescence upconversion material [37] . The addition of NaLuF 4 enables X-ray computed tomography [38] , whereas using NaGdF 4 enables magnetic resonance imaging [39] . To the best of our knowledge, this work presents the first controlled fabrication of sub-50 nm 3D shaped heterogeneous nanocrystals logically programmed by the combinational approaches of OA − -assisted longitudinal growth, transversal growth and selective crystalline facet dissolution with consideration of crystallographic mismatch rates. The nanoscale engineering capability presented in this work enables quantitative studies which are virtually impossible by conventional approaches. We anticipate that optical properties of these nanostructures can be designed to precisely promote or inhibit inter-particle energy transfer. Similarly, magnetic properties may be optimized to enhance magnetic resonance imaging by correlating the morphology with the surface distribution of magnetic signals. In addition, such hybrid nanomaterials may be used as a platform for transporting biologically important molecules across cell membranes. Furthermore, access to a new library of precisely controlled shapes of nanoparticles provide a novel approach for the targeted delivery in nanomedicine where optimized morphologies of these nanoscale molecular carriers will yield greater efficiencies. This process could be further facilitated by harnessing the anisotropic properties of different types of nanoparticles that permit diverse surface functionalizations and multi-modal bio-conjugations. The concept presented in this work may further advance our current capabilities of nanoscale programmable and reproducible engineering of new classes of heterogeneous materials in scalable quantities. Our findings may lead to a new class of multifunctional nanomaterials and provide the groundwork for developing previously unforeseen applications of nanoparticles with complex programmable shapes and surface properties. Hydrothermal synthesis of NaYF 4 crystal The β-NaYF 4 disks were synthesized via a slightly modified hydrothermal reaction. In a typical experiment, NaOH (3.75 mmol) was first dissolved into 1.5 mL of double distilled water, followed by the addition of OA (7.5 mmol) and ethanol (2.5 mL) while undergoing vigorous stirring. Thereafter, an aqueous solution of NaF (0.5 M; 2 mL) was added to form a turbid mixture. Subsequently, a 1.2 mL aqueous solution of YCl 3 (Yb 3+ /Tm 3+ =10/0.5 mol%; 0.2 M) was added and the solution was stirred for 20 min. The resulting mixture was then transferred into a 14 mL Teflon-lined autoclave and heated to 220 °C and the temperature maintained for 12 h. After cooling down to room temperature, the reaction product was isolated by centrifugation and washed with ethanol. In this work, different amounts of NaOH were added to adjust the ratio of OA − /OAH by its reaction with OAH to form OA − . NaYF 4 nanocrystal cores In a typical procedure, 4 ml of methanol solution of YCl 3 (2.0 mmol) was magnetically mixed with OA (38 mmol) and ODE (93 mmol) in a 100-ml three-neck round-bottom flask. The mixture was then degassed under the Ar flow and then heated to 150 °C for 30 min to form a clear solution, before cooling to room temperature. 15 ml of methanol solution containing NH 4 F (8 mmol) and NaOH (5 mmol) was added to the solution of YCl 3 in OA and ODE and stirred for 60 min. The mixture solution was slowly heated to 110 °C and kept at 110 °C for 30 min to completely remove methanol and any residual water. The mixture solution was then quickly heated to the reaction temperature of 300 °C and aged for 1 h. After the solution was left to cool down to room temperature, ethanol was added to precipitate the nanocrystals. The product was washed with cyclohexane, ethanol and methanol for at least 4 times, before the final NaYF 4 nanocrystals were re-dispersed in 10 ml cyclohexane in preparation for their further use. Longitudinal growth of NaYF 4 NRs YCl 3 (0.2 mmol) in 1 ml methanol solution was magnetically mixed with OA (9.5 mmol) and ODE (25 mmol) in a 50-ml three-neck round-bottom flask. The mixture was degassed under Ar flow and heated to 150 °C for 30 min to form a clear solution, and then cooled to room temperature. Methanol solution (5 ml) containing NH 4 F (0.8 mmol) and NaOH (0.5 mmol) was added and stirred for 60 min. The solution was slowly heated to 110 °C and kept at 110 °C for 30 min to completely remove methanol and residual water. The solution was then injected with 0.2 mmol NaYF 4 of nanocrystals in cyclohexane and the mixture kept at 110 °C for another 10 min to evaporate the cyclohexane. Then, the reaction mixture was quickly heated to 310 °C and aged for 1 h. NaGdF 4 /NaYF 4 nano-dumbbells GdCl 3 (0.2 mmol) in 1 ml methanol solution was magnetically mixed with OA (9.5 mmol) and ODE (25 mmol) in a 50-ml three-neck round-bottom flask. The mixture was degassed under an Ar flow and heated to 150 °C for 30 min to form a clear solution, and then cooled to room temperature. Methanol solution (4 ml) containing NH 4 F (0.8 mmol) and NaOH (0.5 mmol) was added to the OA and ODE solution and stirred for 60 min. The solution is slowly heated to 110 °C and kept at 110 °C for 30 min to remove methanol and the remaining water completely. Then, 0.2 mmol of NaYF 4 core nanocrystals in cyclohexane was injected into the reaction solution. After holding the reaction temperature at 110 °C for further 10 min to evaporate all cyclohexane, the reaction mixture was quickly heated to 310 °C and aged for 1 h. NaGdF 4 /NaYF 4 NRs by adding KOH GdCl 3 (0.2 mmol) in 1 ml of methanol solution was magnetically mixed with OA (9.5 mmol) and ODE (25 mmol) in a 50-ml three-neck round-bottom flask. The mixture was degassed under Ar flow and heated to 150 °C for 30 min to form a clear solution, before cooling to room temperature. Methanol solution (5 ml) containing NH 4 F (0.8 mmol), KOH (0.4 mmol) and NaOH (0.5 mmol) was added into the OA and ODE solution and stirred for 60 min. The solution was slowly heated to 110 °C and kept at 110 °C for 30 min to remove the methanol and water completely. The reaction mix was then injected with 0.2 mmol of NaYF 4 core nanocrystals in cyclohexane, into the reaction solution. After holding the reaction mix at 110 °C for further 10 min to evaporate all cyclohexane, the mixture was heated rapidly to 310 °C before aging for 1 h at this temperature. NaYF 4 /NaGdF 4 /NaYF 4 NCs in a bamboo-like shape 0.2 mmol of YCl 3 in 1 ml of methanol solution was magnetically mixed with OA (9.5 mmol) and ODE (25 mmol) in a 50-ml three-neck round-bottom flask. The mixture was degassed under Ar flow and heated to 150 °C for 30 min to form a clear solution, and then cooled to room temperature. Methanol solution (5 ml) containing NH 4 F (0.8 mmol), KOH (0.4 mmol) and NaOH (0.5 mmol) was added into the OA and ODE solution and stirred for 60 minutes. The solution was slowly heated to 110 °C and kept at 110 °C for 30 min to remove the methanol and water completely. The reaction solution was then injected with 0.2 mmol of NaYF 4 /NaGdF 4 NRs in cyclohexane solution. After the reaction at 110 °C for a further 10 min to evaporate all the cyclohexane, the reaction mixture was quickly heated to 310 °C and held at this temperature for 1 h. NaYF 4 /NaGdF 4 /NaYF 4 /NaGdF 4 NCs in a bamboo-like shape The same procedure for synthesizing NaYF 4 /NaGdF 4 /NaYF 4 NCs in bamboo-like shape was repeated, and then followed by the injection of 0.2 mmol of the five-section NaYF 4 /NaGdF 4 /NaYF 4 nano-bamboos which acted as the core, all in cyclohexane solution, into the reaction solution. After holding at 110 °C for a further 10 min to evaporate all cyclohexane, the reaction mixture was quickly heated to 310 °C and held again for 1 h. NaYF 4 /NaGdF 4 /NaNdF 4 NCs in an hourglass shape NdCl 3 (0.4 mmol) in 2 ml of methanol solution was magnetically mixed with OA (9.5 mmol) and ODE (25 mmol) in a 50-ml three-neck round-bottom flask. The mixture was degassed under Ar flow and heated to 150 °C for 30 min to form a clear solution, and then cooled to room temperature. Methanol solution (5 ml) containing KOH (0.8 mmol) and NaOH (0.8 mmol) was added and stirred for 60 min. The solution was slowly heated to 110 °C and kept at 110 °C for 30 min to completely remove the methanol and some of the water. It was then injected with 0.1 mmol 50 nm × 60 nm NaYF 4 /NaGdF 4 nano-prisms particles, in a solution of cyclohexane. After having been kept at 110 °C for another 10 min to evaporate all cyclohexane, the reaction mixture was quickly heated to 310 °C. Samples (500 ul) of the reaction solution were collected each time with a syringe at 5, 15, 30, 40, 50 and 60 min after the start of the reaction. Transversal growth of NaGdF 4 shell onto NaYF 4 core GdCl 3 (0.1 mmol) in 1 ml methanol solution was magnetically mixed with OA (19.0 mmol) and ODE (18.7 mmol) in a 50-ml three-neck round-bottom flask. The mixture was degassed under Ar flow and heated to 150 °C for 30 min to form a clear solution, and then cooled to room temperature. Methanol solution (3 ml) containing NH 4 F (0.4 mmol) and NaOH (0.15 mmol) was added into the OA and ODE solution and stirred for 60 min. The solution was slowly heated to 110 °C and kept at 110 °C for 30 min to remove completely the methanol and water. Then 0.1 mmol of the NaYF 4 cores in cyclohexane solvent were injected into the reaction mix. After being kept at 110 °C for further 10 min to evaporate all cyclohexane, the reaction mixture was quickly heated up to 290 °C and held at that temperature for 3 h. Synthesis of NaYF 4 /NaGdF 4 /NaNdF 4 NCs in flower shape NdCl 3 (0.1 mmol) in 1 ml of methanol solution was magnetically mixed with OA (19 mmol) and ODE (18.7 mmol) in a 50-ml three-neck round-bottom flask. The mixture was degassed under Ar flow and heated to 150 °C for 30 min to form a clear solution, and then cooled to room temperature. Methanol solution (5 ml) containing NaOH (0.6 mmol) was added and stirred for 60 min. The solution was slowly heated to 110 °C and kept at 110 °C for 30 min to completely remove the methanol and some of the water. Then, the reaction mix was injected with 0.1 mmol of 50 nm NaYF 4 /NaGdF 4 nano-prisms prisms (NaGdF 4 growing on the lateral faces of NaYF 4 nanocrystal), suspended in a cyclohexane solution. After holding at 110 °C for another 10 min to evaporate all cyclohexane, the reaction mixture was quickly heated to 300 °C. samples (500 ul) of the reaction solution were collected each time with a syringe after 10, 25 and 45 min of the reaction time. Synthesis of NaYF 4 /NaGdF 4 /NaNdF 4 sharp-end dumbbell NdCl 3 (0.1 mmol) in 1 ml of methanol solution was magnetically mixed with OA (9.5 mmol) and ODE (25 mmol) in a 50-ml three-neck round-bottom flask. The mixture was degassed under Ar flow and heated to 160 °C for 30 min to form a clear solution, and then cooled to room temperature. Methanol solution (5 ml) containing KOH (0.2 mmol) and NaOH (0.2 mmol) was added and stirred for 60 min. Note: in this reaction no NH 4 F was added to the solution. The solution was slowly heated to 110 °C and kept at 110 °C for 30 min to remove the methanol and the water completely. It was then injected with 0.1 mmol of NaYF 4 /NaGdF 4 NR particle in suspended in cyclohexane solvent into the reaction solution. After holding at 110 °C for a further 10 min to evaporate all cyclohexane, the reaction mixture was quickly heated to 310 °C and held at this temperature for a further 30 min. Synthesis of NaYF 4 /NaGdF 4 /NaNdF 4 round-end dumbbell NdCl 3 (0.1 mmol) in 1 ml of methanol solution was magnetically mixed with OA (9.5 mmol) and ODE (25 mmol) in a 50-ml three-neck round-bottom flask. The mixture was degassed under Ar flow and heated to 160 °C for 30 min to form a clear solution, and then cooled to room temperature. Methanol solution (5 ml) containing NH 4 F (0.3 mmol), KOH (0.2 mmol) and NaOH (0.2 mmol) was added and the mixture was stirred for 60 min. The solution was slowly heated to 110 °C and kept at 110 °C for 30 min to remove the methanol and the water completely. Then, it was injected with 0.1 mmol of NaYF 4 /NaGdF 4 NRs suspended in cyclohexane into the reaction solution. After being held at 110 °C for further 10 min to evaporate all cyclohexane, the reaction mixture was quickly heated to 310 °C and held for 30 min at this temperature. Synthesis of pure α -NaGdF 4 NCs Methanol solution (2 ml) of GdCl 3 (1.0 mmol) was magnetically mixed with OA (19 mmol) and ODE (47 mmol) in a 100-ml three-neck round-bottom flask. The mixture was degassed under Ar flow and heated to 150 °C for 30 minutes to form a clear solution, and then cooled to room temperature. Methanol solution (10 ml) containing NH 4 F (4 mmol) and NaOH (2.5 mmol) was added and stirred for 60 min. Then, the solution was slowly heated to 110 °C and kept at 110 °C for 30 min to remove the methanol and water completely. After that, the reaction mixture was quickly heated to 240 °C and aged for 45 min. Synthesis of NaLuF 4 /NaYF 4 NRs LuCl 3 (0.1 mmol) in 1 ml method solution was magnetically mixed with OA (19 mmol) and ODE (25 mmol) in a 50-ml three-neck round-bottom flask. The mixture was degassed under Ar flow and heated to 150 °C for 30 min to form a clear solution, and then cooled to room temperature. Methanol solution (2 ml) containing NaOH (0.15 mmol) and 0.4 mmol NH 4 F was added and stirred for 60 min. The solution was slowly heated to 110 °C and kept at 110 °C for 30 min to completely remove the methanol and some of the water. It was then injected with 0.4 mmol of NaYF 4 seed particles in a cyclohexane solution. After holding the reaction mix at 110 °C for a further 10 min to evaporate cyclohexane, the reaction mixture was quickly heated to 290 °C and held at that temperature for a further 1 h. Synthesis of NaLuF 4 /NaYF 4 NRs with NaGdF 4 double-ring GdCl 3 (0.1 mmol) in 1 ml methanol solution was magnetically mixed with OA (19.0 mmol) and ODE (18.7 mmol) in a 50-ml three-neck round-bottom flask. The mixture was degassed under Ar flow and heated to 150 °C for 30 min to form a clear solution, and then cooled to room temperature. Methanol solution (2 ml) containing NaOH (at 0.15 mmol) was added and stirred for 60 min. The solution was slowly heated to 110 °C and kept at 110 °C for 30 min to completely remove the methanol and some of the water. It was then injected with 0.1 mmol of the NaYF 4 /NaLuF 4 seed particles, in a cyclohexane solution, into the reaction solution. After having been held the reaction mix at 110 °C for another 10 min to evaporate cyclohexane, the reaction mixture was quickly heated to 300 °C. It was then, injected with 0.02 mmol of α -NaGdF 4 nanocrystals into the reaction system. This was done every 10 min for 5 times at 300 °C. The reaction mix was held at this temperature for another 10 min after the last injection. How to cite this article: Liu, D. et al . Three-dimensional controlled growth of monodisperse sub-50 nm heterogeneous nanocrystals. Nat. Commun. 7:10254 doi: 10.1038/ncomms10254 (2016).